Ultrafast universal quantum control of a quantum-dot charge qubit using Landau–Zener–Stückelberg interference A basic requirement for quantum information processing is the ability to universally control the state of a single qubit on timescales much shorter than the coherence time. Although ultrafast optical control of a single spin has been achieved in quantum dots, scaling up such methods remains a challenge. Here we demonstrate complete control of the quantum-dot charge qubit on the picosecond scale. We observe tunable qubit dynamics in a charge-stability diagram, in a time domain, and in a pulse amplitude space of the driven pulse. The observations are well described by Landau–Zener–Stückelberg interference. These results establish the feasibility of a full set of all-electrical single-qubit operations. Although our experiment is carried out in a solid-state architecture, the technique is independent of the physical encoding of the quantum information and has the potential for wider applications. Universal single-qubit gates are key elements in a quantum computer, as they provide the fundamental building blocks for implementing complex operations [1] , [2] , [3] . In the standard circuit model, arbitrary single-qubit rotations [1] , together with two-qubit controlled-NOT gates, provide a universal set of gates. In the alternative measurement-based models, such as the one-way quantum computer, the ability to carry out single-qubit operations from the source of a specific multi-particles state can generate every possible quantum state [2] and offer practical algorithms. Additionally, with only single-qubit operations and teleportation, one can construct a universal quantum computer [3] . In the Bloch sphere model of qubit states, a universal single-qubit gate requires arbitrary rotations around at least two axes. The charge [4] , [5] or spin [6] , [7] , [8] , [9] degrees of freedom of an electron in quantum dots are particularly attractive for the implementations of qubits. Owing to the fast charge or spin decoherence times in semiconductor quantum dots, which are typically less than a few nanoseconds [4] , [5] , [6] , [7] , [8] , [9] , control operating on the picosecond timescale may be necessary. Until now, ultrafast manipulations of a single qubit in quantum dots have been performed using pulsed laser fields [10] , [11] , [12] . Alternatively, electrical pulses can be generated much more easily by simply exciting a local electrode. Logic gate operations and readouts can be carried out all-electrically, much like those in current mainstream semiconductor electronics. Additionally, this all-electric technique provides a simple pathway for greater spatial selectivity to locally address the individual qubits and remove obstacles to scalability. Therefore, universal electrical control on a picosecond scale is highly desirable to allow coherence to be maintained during the completion of a large number of operations. Over the last few decades, the Landau–Zener–Stückelberg (LZS) interference has served as a textbook model for quantum phenomena [13] , that occurs when a system sweeps through the anti-crossing of two energy levels. LZS has also gained particular interest for quantum control [8] , [14] because it is less sensitive to certain types of noise and might enable the implementation of a universal gate with high fidelity [15] , [16] , [17] . Here we experimentally demonstrate such a scheme for a single-charge qubit in a double quantum dot (DQD), using a single pulse. We may add that very recently LZS interference has been observed under a continuous microwave driving, in both an electrostatic-defined [18] and a donor-based [19] semiconductor DQD systems. 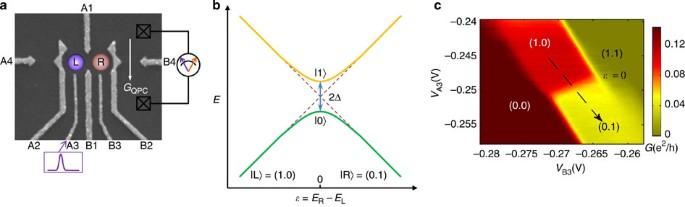Figure 1: Experimental set-up to characterize, control and measure single-electron charges. (a) Scanning electron micrograph of the confinement gates that defined the DQD and the QPC charge-sensing channel. The two dots have a lithographic dimension of ~300 nm. (b) Energy diagram of the DQD charge qubit. The green and yellow solid lines represent the energy levels for the bonding and anti-bonding states, respectively. With a finite inter-dot coupling, the lines are anti-crossed near the resonance point. (c) Colour scale plot of the charge-sensing signal as a function of the gate voltagesVA3andVB3. The notation (n,m) represents the effective left and right dot occupancy. Charge qubit in a DQD Figure 1a provides a scanning electron micrograph of the sample used in the experiments, in which the metal gate pattern electrostatically defines a DQD and a nearby quantum point contact (QPC) detector within a GaAs/AlGaAs heterostructure. All measurements were conducted in a dilution refrigerator equipped with high-frequency lines (details of sample structures and experimental techniques are given in the Methods section). A single-electron charge in the DQD is used to encode the charge qubit [4] , [5] , [20] . An excess valence electron in the left and right dots defines the basis states |L and |R , respectively. The schematic diagram in Fig. 1b illustrates that the energies of the qubit states can be continuously tuned by the level detuning ε = E R − E L , in which E L and E R are the energy levels for the electron in the left and right dots for an uncoupled DQD, respectively. In the presence of inter-dot tunnelling that couples two dots, a characteristic anti-crossing occurs between the two-qubit levels near the resonance ( ε =0). For our experiments, the anti-crossing gap 2Δ is adjusted to 20.7 μeV, which corresponds to a Rabi frequency of 5.0 GHz. We have experimentally determined the Rabi frequency from the coherent oscillations excited by a square, non-adiabatic pulse as shown in Supplementary Fig. S1b . We denote the ground and excited states as |0 and |1 , which are roughly the charge eigenstates far from the resonance. Figure 1: Experimental set-up to characterize, control and measure single-electron charges. ( a ) Scanning electron micrograph of the confinement gates that defined the DQD and the QPC charge-sensing channel. The two dots have a lithographic dimension of ~300 nm. ( b ) Energy diagram of the DQD charge qubit. The green and yellow solid lines represent the energy levels for the bonding and anti-bonding states, respectively. With a finite inter-dot coupling, the lines are anti-crossed near the resonance point. ( c ) Colour scale plot of the charge-sensing signal as a function of the gate voltages V A3 and V B3 . The notation ( n , m ) represents the effective left and right dot occupancy. Full size image The characterization of the system is shown in the charge-stability diagram for the DQD ( Fig. 1c ), which integrates the few-electron regime so that ~2–3 electrons occupy each dot (for the full diagram, see Supplementary Fig. S1a ). Our experiments are performed for a variety of charge states. As they contain identical physics, for consistency, we present only the data collected from one charge configuration. The system can be conveniently described in a valence electron number configuration that consists of four relevant charge states: (0,0), (1,0), (0,1) and (1,1). A prominent boundary can be observed between (1,0) and (0,1) and marks the inter-dot transition line corresponding to the ε =0 resonance. Observations of LZS interference Our scheme to control a single-charge qubit using a Gaussian-shaped short pulse is shown in Fig. 2a . The system is initially prepared in the |R state at a positive detuning ε 0 , which is far from the resonance. During the rising phase of the pulse, the sweeping pulse takes the system adiabatically to the anti-crossing point at t = t 1 at which a significant probability exists for a non-adiabatic transition to the excited state |1 . 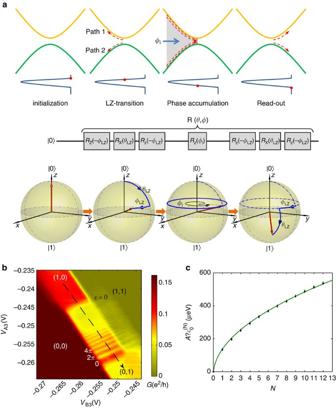Figure 2: Experimental demonstration of theRxandRzoperations via the LZS interference. (a) Illustration of the LZS interference evolution in the four different time stages of the driven pulses, indicated by the solid dots. The diagrams in the below schematically illustrate the circuits for unitary transformations on one qubit and the resulting evolution of the qubit trajectories on the Bloch sphere. The bracket highlights the decomposition of the arbitrary single-qubit operation. (b) Under a short driven pulse, the charge-stability diagram inFig. 1chas been largely altered and a sequence of additional lines has emerged. (c) The construction interference finger locationsε0(N)(dots) along the line in (b) as a function of the interference orderN. The error bars are determined from the least-squares fit to the data. The solid line is obtained from a theoretical expression. This probability is the Landau–Zener transition represented by the following formula: Figure 2: Experimental demonstration of the R x and R z operations via the LZS interference. ( a ) Illustration of the LZS interference evolution in the four different time stages of the driven pulses, indicated by the solid dots. The diagrams in the below schematically illustrate the circuits for unitary transformations on one qubit and the resulting evolution of the qubit trajectories on the Bloch sphere. The bracket highlights the decomposition of the arbitrary single-qubit operation. ( b ) Under a short driven pulse, the charge-stability diagram in Fig. 1c has been largely altered and a sequence of additional lines has emerged. ( c ) The construction interference finger locations ε 0 ( N ) (dots) along the line in ( b ) as a function of the interference order N . The error bars are determined from the least-squares fit to the data. The solid line is obtained from a theoretical expression. Full size image in which υ is the sweep velocity of the driven pulse through the anti-crossing point. As the pulse takes the system further past ε =0, two different trajectories at different energies can coherently interfere. Upon returning to ε =0 at t = t 2 , the two trajectories, caused by the coherent interference, have also accumulated a phase difference of magnitude A projective read-out is performed at the end of the pulse to measure the |L state for a constructive interference and the |R state for a destructive interference, known as the LZS interference. Thus, the LZS process consists of both the non-adiabatic level transition and the adiabatic phase accumulation. The Bloch sphere model provides a convenient picture to understand the quantum control of a charge qubit. Using this model, the charge state is represented as a vector, in which the ground and excited states |0 and |1 are at the north and south poles, respectively. In this model, the dynamics of the qubit can be represented by applying the appropriate sequence of unitary operation matrices to the initial state. The matrices give rise to a rotation on the Bloch sphere around the x axis by an angle θ and around the z axis by an angle φ . At a Landau–Zener transition, the initial state becomes a coherent superposition of |1 and |0 with a phase φ LZ related to the Stokes phenomenon [13] . The relative amplitudes of |1 and |0 depend on P LZ . This behaviour corresponds to the transformation R z (− φ LZ ) R x ( θ LZ ) R z (− φ LZ ), seen as successive x and z -rotations (see the Supplementary Discussion for details), and θ LZ =2 sin −1 √ P LZ . In the phase accumulation stage, the qubit undergoes a single rotation about the z axis, referred to as the phase-shift gate operation R z ( φ i ). Thus, the combination of R x and R z enables arbitrary one-qubit rotations R ( θ , φ ) on the Bloch sphere and the LZS pulse rotates the input state on the Bloch sphere to the output state as illustrated in Fig. 2a . The coherent control of our charge qubit is evident in the stability diagram ( Fig. 2b ), which is considerably altered as compared with that without an applied pulse. We observe many additional lines parallel to the inter-dot transition line. These additional lines are a signature of the excitation of the LZS interference by the pulse. In our device, the right barrier to the bath is slightly more open than the left barrier, and one can observe that the charge-addition lines (0,0)—(1,0) and (0,1)—(1,1) are less visible. As a result, an interesting triangular-shaped area exists in which the electron has a high probability of escaping to the reservoir before the inter-dot transition is completed. The additional lines in Fig. 2b can be easily understood. For the line labelled 0, the pulse takes the system just past the anti-crossing point. At the next line, the pulse can take the qubit further, passing ε =0 and accumulating a total phase of 2 π . Therefore, the lines represent the constructive interference fringes between the successive Landau–Zener transitions that correspond to an accumulated total phase of 2 πN . To confirm our identification, we have derived an analytical expression for the locations, ε 0 ( N ) , of the constructive interference fingers for a triangular pulse [21] . The triangular pulse is a simple approximation of the actual Gaussian profile of our pulse and can readily yield an intuitive analytical expression (see the Supplementary Discussion ), , in which A is the pulse amplitude with units of energy that can be converted from voltage using the lever-arm conversion factor and t r is the pulse-raising time. Figure 2c compares the experimental finger positions with a theoretical curve obtained using the above equation, and reasonable agreement can be achieved. Complete and ultrafast quantum control of the charge states The ability to fully control the charge qubit is also studied using the LZS interference patterns. Controlling the amplitude of the driven pulse while the time profile of the pulse is fixed sets the speed υ of the passage through the anti-crossing point, thus the R x ( θ LZ ) rotation angle θ LZ and the R z ( φ LZ ) rotation angle φ LZ . Tuning the pulse time interval in the phase accumulation stage sets the R z ( φ i ) rotation angle φ i . The parameters θ LZ , φ LZ and φ i are sufficient to rotate the input qubit to any point on the Bloch sphere, or more generally, to implement a universal one-qubit operation R ( θ , φ ) using the LZS pulse profile [22] , [23] . To demonstrate the ability of the LZS method to generate tunable unitary transformations, we use the amplitude of the driven source as a control parameter. The charge state probability P |L› as a function of the qubit detuning position ε 0 and the voltage amplitude A under a 150-ps short pulse is provided in Fig. 3a . Given the detuning and driven pulse amplitude, such interference patterns exhibit fringes that rise again from the constructive interference between successive Landau–Zener transitions at φ as a multiple of 2 π . A characteristic of the LZS driving occurs when the z -rotations result in the total phase φ =2 πN ; the total x -rotation angle θ is generally maximized as 2 θ LZ , which increases monotonically with the driven amplitude (see Supplementary Discussion for details). We verify this result by extracting the total rotation angles ( θ , φ ) of the Bloch vector from Fig. 3b (a horizontal cut at ε 0 =400 μeV of Fig. 3a ) as it undergoes LZS interference. These rotation angles are also parametrically plotted in Fig. 3c , demonstrating the expected behaviour as a function of the pulse amplitude. In addition, we note that the fit of φ is better than that of θ , indicating that the phase-shift gates have higher intrinsic resistance to certain decoherence [15] , [16] . These findings suggest that the LZS pulse amplitude should be an important tuning parameter for optimizing the quantum control of two-level systems. 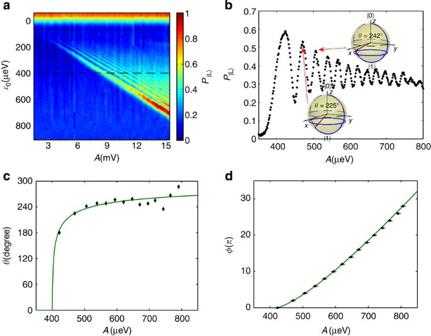Figure 3: Arbitrary single-qubit rotationsR(θ,φ) with a controlled LZS interference amplitude. (a) The probability of the qubit in the |Lstate as a function of the energy positionε0and the driven pulse amplitudeA. (b) Charge state probabilityP|L›along the line inFig. 3a. The reconstructed evolution of the Bloch vector for two interference nodes is also labelled. (c,d) Total rotation anglesθaround thexaxis andφaround thezaxis (dots) of the Bloch sphere were extracted from the data shown inFig. 3b, as a function of the controlled pulse amplitude. The error bars are determined from the least-squares fit to the data. The solid lines are theoretical predictions. Figure 3: Arbitrary single-qubit rotations R ( θ , φ ) with a controlled LZS interference amplitude. ( a ) The probability of the qubit in the |L state as a function of the energy position ε 0 and the driven pulse amplitude A . ( b ) Charge state probability P |L› along the line in Fig. 3a . The reconstructed evolution of the Bloch vector for two interference nodes is also labelled. ( c , d ) Total rotation angles θ around the x axis and φ around the z axis (dots) of the Bloch sphere were extracted from the data shown in Fig. 3b , as a function of the controlled pulse amplitude. The error bars are determined from the least-squares fit to the data. The solid lines are theoretical predictions. Full size image The LZS interferences are further studied in the time-domain. We use a low-pass filter to shape the time-varying, square-driven pulse into an approximately Gaussian profile for the investigations. 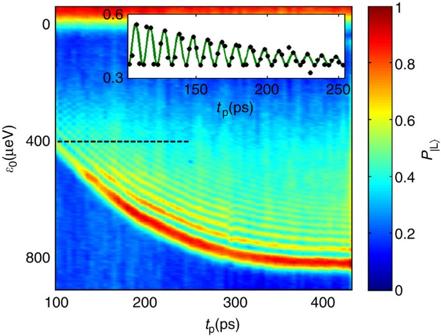Figure 4: Rotation dynamics of the LZS interference. The occupation of the qubit in the |Lstate as a function of the energy positionε0and pulse lengthtp. The pulse is shaped using a 2.7-GHz low-pass filter. The inset shows a line cut revealing clear, ultrafast oscillations as a function of time. Figure 4 shows the charge state occupation P |L› as a function of both the detuning energy position ε 0 and the pulse width t p . Up to 10 LZS interference fringes can be clearly observed. The brightest line in the figure can be understood as the detuning pulse precisely at the anti-crossing point, and the subsequent finer lines corresponds to full phase accumulations of 2 π , 4 π and so on. We also simulate the evolution of the charge qubit by numerically solving the master equations as described in the Supplementary Discussion . This simulation (as shown in Supplementary Fig. S2 ) is in reasonable agreement with the experimental data. In particular, fast time-evolutions are observed in the insert of Fig. 4 . For example, at a detuning energy of ε 0 =400 μeV, only ~10 ps is required to accumulate a phase of 2 π that corresponds to a full cycle of R z operations of the qubit. For gate defined GaAs qubits, the phase rotation time can be electrically manipulated at this time scale. Figure 4: Rotation dynamics of the LZS interference. The occupation of the qubit in the |L state as a function of the energy position ε 0 and pulse length t p . The pulse is shaped using a 2.7-GHz low-pass filter. The inset shows a line cut revealing clear, ultrafast oscillations as a function of time. Full size image To further highlight the importance of the LZS interference for a general single-qubit gate, we consider the following example: Tuning the speed of passage to yield P LZ =1/2, the total rotation is a Hadamard gate with an arbitrary phase [22] . As the Rabi frequency can be reliably tuned to 10 GHz, the total rotation can be completed in ~50 ps. Decoherence information in the amplitude spectroscopy Decoherence of the qubit due to its environment can be readily extracted from the amplitude spectroscopy [24] , [25] (for details, see the Supplementary Discussion ). It is useful to evaluate the Fourier transform of the occupation probability in which k A and k ε represent the reciprocal-space variables corresponding to the real-space variables A and ε , respectively. The two-dimensional Fourier transform of the data in Fig. 3a is provided in Fig. 5 . 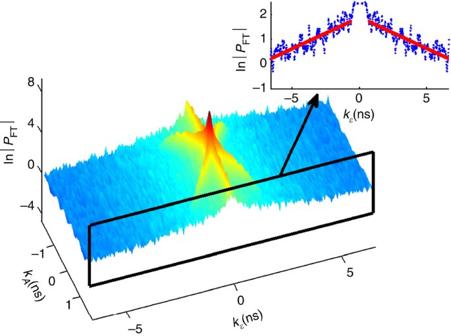Figure 5: Coherence information displayed in the amplitude spectroscopy of the LZS interference. Discrete Fourier transform of the experimental spectroscopy triangle inFig. 3a. The three-dimentional plot of the Fourier intensity was used to extract the intrinsic dephasing timeT2and the ensemble averagingT2* from the exponential decay (the red line in the inset is a fit, see the main text). The reciprocal-space variableskAandkεcorrespond to the real-space variablesAandε, respectively. As k ε is practically a timescale, decoherence leads to an attenuation in the k ε direction as follows [25] : Figure 5: Coherence information displayed in the amplitude spectroscopy of the LZS interference. Discrete Fourier transform of the experimental spectroscopy triangle in Fig. 3a . The three-dimentional plot of the Fourier intensity was used to extract the intrinsic dephasing time T 2 and the ensemble averaging T 2 * from the exponential decay (the red line in the inset is a fit, see the main text). The reciprocal-space variables k A and k ε correspond to the real-space variables A and ε , respectively. Full size image Therefore, both the intrinsic dephasing time T 2 and the inhomogeneous broadening T 2 * can be extracted from the overall amplitude decay. One must emphasize that this amplitude spectroscopy has an advantage over the two types of dephasing times because T 2 and T 2 * exhibit different k ε dependences. In our data, the Fourier intensity, three-dimensionally plotted in a log scale, is apparently dominated by a linear k ε dependence. Therefore, T 2 is extracted without requiring spin-echo experiments. A typical trace form Fig. 5 yields an estimation of T 2 =4±0.6 ns, while T 2 * is difficult to extract as the quadratic term is relatively small and is masked by noise. Nevertheless, the T 2 decoherence time is much longer than the 10 ps required for a 2 π phase rotation. The decoherence and relaxation times can greatly effect the single-qubit operation fidelity as shown in Supplementary Fig. S3 . In summary, we have used a shaped electrical pulse to create LZS interference in a semiconductor DQD charge qubit. The LZS interference-induced x -rotation operations along with the dynamic phase-gate operations can form a basis for rapid, universal, all-electric one-qubit gate operations in a few tens of picoseconds. These results represent progress towards the implementation of semiconductor quantum dot-based qubits. Our results are an important addition to the rapidly growing toolbox of quantum information processing because they are generally applicable to systems that avoid crossings, including both artificial and natural two-level systems. This well-controlled, solid-state system could also be seen as an analogue quantum simulator of a real atom undergoing LZS interferometry [26] . A similar timescale for electrical control was also observed in ref. 27 in a quantum-dot charge qubit using non-adiabatic voltage pulses. Devices The DQD device is defined by electron beam lithography on a molecular beam epitaxially grown GaAs/AlGaAs heterostructure. The two-dimensional electron gas is located 95 nm below the surface. The two-dimensional electron gas has a density of 3.2 × 10 11 cm −2 and a mobility of 1.5 × 10 5 cm 2 V −1 s −1 . Figure 1a provides the scanning electron micrograph of the surface gates. Six gates—A1, A2, A3, B1, B2 and B3—shape the DQD. Gates B4 and B2 form a QPC charge-sensing channel for counting the DQD electron occupations via capacitive coupling. Control and measurements The experiments were performed in an Oxford Triton dilution refrigerator with a base temperature of 30 mK. An Agilent 81134A pulse generator with a time resolution of 1 ps was used to deliver fast pulse trains through semi-rigid coaxial transmission lines to the A3 side gate of the device. The conductance through the QPC, G QPC , depends on the change in local charge configuration and provides a sensitive metre for the number of electrons in the left and right dots. The charge state probability is determined by normalizing the charge sensor conductance to the adjacent plateaus in the charge-stability diagram. This measurement technique has been reportedly used in single-charge qubits and offers the experimental convenience of integrating initialization, manipulation and measurement in the same pulse [7] . In our experiment, a pulse repetition rate of 30 MHz was chosen to ensure that the qubit is relaxed to the initial state and to carry out a sufficient number of projective measurements (~10 7 times) for an adequate signal-to-noise ratio. The ensemble averaging of these measurements, in terms of the average charge detector conductance, allows us to directly obtain the probability of the qubit states. How to cite this article: Cao, G. et al. Ultrafast universal quantum control of a quantum-dot charge qubit using Landau–Zener–Stückelberg interference. Nat. Commun. 4:1401 doi: 10.1038/ncomms2412 (2013).